Strong bias in the bacterial CRISPR elements that confer immunity to phage Clustered regularly interspaced short palindromic repeats (CRISPR)–Cas systems provide adaptive immunity against phage via spacer-encoded CRISPR RNAs that are complementary to invasive nucleic acids. Here, we challenge Streptococcus thermophilus with a bacteriophage, and used PCR-based metagenomics to monitor phage-derived spacers daily for 15 days in two experiments. Spacers that target the host chromosome are infrequent and strongly selected against, suggesting autoimmunity is lethal. In experiments that recover over half a million spacers, we observe early dominance by a few spacer sub-populations and rapid oscillations in sub-population abundances. In two CRISPR systems and in replicate experiments, a few spacers account for the majority of spacer sequences. Nearly all phage locations targeted by the acquired spacers have a proto-spacer adjacent motif (PAM), indicating PAMs are involved in spacer acquisition. We detect a strong and reproducible bias in the phage genome locations from which spacers derive. This may reflect selection for specific spacers based on location and effectiveness. Host–parasite interactions and co-evolution are critical in a wide range of ecological and evolutionary processes. They shape microbial population structure, speciation and the evolution of diversity, impact mutation fixation rates, influence the ecology of pathogen virulence [1] , [2] and affect the probability of lineage extinction. Given their biosphere and technological importance, the interactions of microorganisms with the viruses that replicate within them are of special interest. To enable coexistence with their viruses, bacteria and archaea have evolved a variety of resistance mechanisms, including prevention of phage adsorption, the inhibition of DNA injection, restriction-modification systems and abortive infection systems [3] , [4] , [5] , [6] . Recent research, first described in 2002, has demonstrated the importance of a novel adaptive mechanism that provides bacteria immunity to phage [7] , [8] , that is based on clustered regularly interspaced short palindromic repeats (CRISPR) loci and their associated genes ( cas ) [9] , [10] , [11] . CRISPR–Cas immunity involves a multistep process that begins with the acquisition of short, exogenous nucleic acid fragments called spacers. CRISPR locus transcription generates an RNA that is loaded onto a ribonucleoprotein Cas complex, which cleaves the matching exogenous nucleic acid (interference) [12] . The biochemistry of interference has been extensively studied [12] , [13] , [14] , but spacer acquisition, is not well understood. Short conserved proto-spacer adjacent motifs (PAMs) flanking the spacer target on the phage genome have been shown to be required for silencing of invading elements, but their role in spacer acquisition remains unclear [12] , [15] , [16] , [17] . Further, little is known about how the viral genome is sampled by the Cas proteins, whether certain fragments may be preferentially acquired or selected for, or of the dynamics of phage–host genome co-evolution. Here, we challenged S. thermophilus DGCC7710 [9] , [18] , [19] , [20] with lytic phage D2972 [21] and monitored CRISPR locus expansion in the bacterial population daily over 15 days (100 generations). In contrast to prior research, where shallow sequencing of the CRISPR locus was used to demonstrate spacer acquisition [18] , we used 454-sequencing of PCR-amplicons to monitor the expanding CRISPR loci at the leader end. The deep sampling afforded by this approach allowed us to test for bias in the spacer complement, both in terms of spacer representation and target region on the phage genome, to evaluate the importance of the PAM for spacer acquisition, and to track population fluctuations. The research required development of bioinformatics tools to recover and classify spacer sequences and to reconstruct locus geometry. Locus geometry reconstruction allowed us to separate the effects of proliferation of spacers due to increase in relative abundance of host strains from high spacer abundance due to insertion of the same spacer in multiple incorporation events. We conducted two independent experiments with phage:host ratios (multiplicity of infection, MOI) of 2:1 and 10:1, and targeted the two active CRISPR loci, CRISPR1 and CRISPR3, both type II-A CRISPR–Cas systems [22] . The repeatable unexpected bias in the spacer acquisition observed in this work combined with the large amount of data processed reveals further insight into this CRISPR-Cas system step. CRISPR spacer deep-sequencing Overall, we recovered 443,871 newly acquired spacer sequences from 554,803 sequencing reads from three experimental series, across 15 daily samples ( Supplementary Table S1 ). Spacers sharing 80% sequence identity over 80% of their length were grouped into spacer types to avoid artifacts due to sequencing error ( Supplementary Fig. S1 and Computational analyses in Methods). Phage and host numbers were similar in the two independent experiments with phage:host ratios of 2:1 and 10:1, that targeted the two active CRISPR loci experiments, and remained fairly constant, except for a dramatic decline and recovery between days 3 and 5 ( Fig. 1 ). 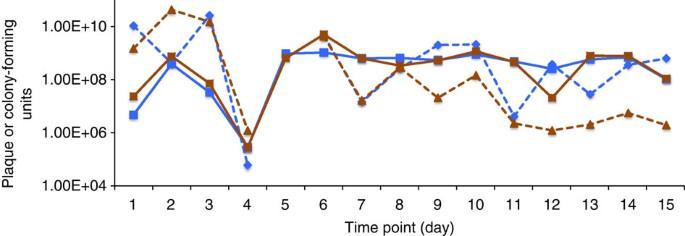Figure 1: Dynamics of host–phage co-existence and co-evolution. The fluctuations in the number of plaque- (dashed lines) or colony- (straight lines) forming units in the MOI2 (blue) and MOI10 (brown) experiments are shown across 15 days. Figure 1: Dynamics of host–phage co-existence and co-evolution. The fluctuations in the number of plaque- (dashed lines) or colony- (straight lines) forming units in the MOI2 (blue) and MOI10 (brown) experiments are shown across 15 days. Full size image Sampled spacers are associated with PAMs A PAM, AGAAW, previously reported for CRISPR1 [18] , [20] was identified in the direct vicinity of 95.19% of the overall spacer sampled ( Supplementary Table S2 ). Interestingly, that perfect motif was associated with only 45.85% of the unique phage targets, although single, double or triple single-nucleotide polymorphisms (SNPs) accounted for 85.5%, 95.6% and 98.5%, of the unique PAMs, respectively ( Fig. 2 ). Given that extremely deep-sequencing at relatively closely spaced time points captures cells throughout their life cycle and not just those cells that survive and proliferate, this result indicates that a PAM is important for spacer acquisition although imperfect PAMs may be sampled. The perfect AGAAW motif oversampling, might indicate increased efficiency for CRISPR-mediated interference. Likewise, PAM polymorphism may reflect flexibility in the biochemical processes that drive crRNA-mediated interference. 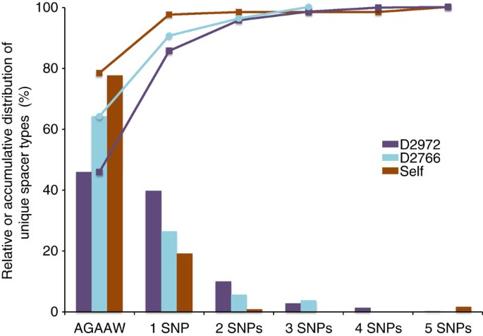Figure 2: Single-nucleotide polymorphisms in PAMs. Relative (bars) and accumulative (lines) distribution of CRISPR1 PAM for unique spacer types that target phage D2972, phage D2766, and self targetS. thermophilusgenome. Figure 2: Single-nucleotide polymorphisms in PAMs. Relative (bars) and accumulative (lines) distribution of CRISPR1 PAM for unique spacer types that target phage D2972, phage D2766, and self target S. thermophilus genome. Full size image Sensitivity of the approach and support of PAM importance Of all the unique spacer types sequenced, 1.23% uniquely matched to D2766, a phage closely related to D2972. Likewise, 64.2% of the unique D2766 proto-spacers had an AGAAW PAM (allowing for one or two SNPs in the PAM, this increased to 90.5% and 96.2%, respectively). The high incidence of PAMs associated with proto-spacers in D2766 further supports both the involvement of this motif in spacer acquisition and the tolerance for some polymorphism in the PAM ( Fig. 2 ). Based on the number of incorporation events involving spacers unique to each phage, we infer that phage D2972 was 35 times more abundant than D2766 (having a ratio of number of independent events of unique spacer types to each phage, of 7:1; Supplementary Table S3 ). Autoimmunity is rare and lethal Surprisingly, we observed acquisition of 120 spacer types (representing 0.04% of the 443,871 sampled spacers) matching the host chromosome, including 117 perfect matches, 78.33% of which were associated with a perfect AGAAW PAM (97.5% allowing for one SNP in the PAM). We investigated the incidence of this phenomenon by distinguishing independent events in which spacers were sampled from the host chromosome. Incorporation events were defined when one specific spacer type was flanked by different spacers. The average number of events for self-targeting spacer types was 1.01 with a spacer frequency of 1.36, indicating that autoimmunity generates unstable and likely non-viable genotypes. This reflects an imperfect ability of the host to differentiate self from non-self [23] and indicates strong selection against cells that acquire self-targeting spacers, presumably because self-targeting spacers are lethal. Selection of spacers shows unexpected bias There are 233 candidate proto-spacers that can be theoretically acquired from D2972 into CRISPR1 (AGAAW PAM, frequency of 95.19%), and 483 into CRISPR3 (GGNG PAM, frequency of 96.68%) [19] . In both experiments, we noted that some specific CRISPR1 and CRISPR3 spacers were highly represented in the set of newly acquired spacers. More importantly, we found that 9 of the 20 most frequently sampled CRISPR1 spacers were shared between the two experiments (MOI2 and MOI10; Supplementary Table S4 ). Similarly, 9 of the 20 most highly sampled CRISPR3 spacers also were shared in the two experiments. Statistical analysis based on probability revealed that this is a non-random over-sampling of a subset of the proto-spacer pool ( e- values of ~1 × 10 −9 and ~1 × 10 −11 for CRISPR1 and CRISPR3, respectively). For the MOI2 experiment, we identified the 10 most abundant newly acquired CRISPR1 spacers in the bacterial population at each of the 15 time points. When combined, this group includes only 27 spacer sequences, and accounts for between 82% and 99% of all spacers sampled on any individual day ( Fig. 3 ). Similarly, for the MOI10 experiment, only 35 CRISPR1 spacer types represented between 82% and 99% of the spacers across the fifteen time points ( Supplementary Fig. S2 ). Analysis of day-to-day variation (sum of the changes in spacer frequency between consecutive days) revealed between 4.5% and 58.8% daily spacer turnover (average 23%) in the MOI2 experiment and between 14.3% and 53.9% daily turnover (average 28%) in the MOI10 experiment. The most dramatic changes occurred in the first 4 days for both experiments, coinciding with the time period with the highest fluctuations of bacterial and phage abundances ( Fig. 1 ). A similar trend was observed for the CRISPR3 locus ( Supplementary Fig. S3 ). 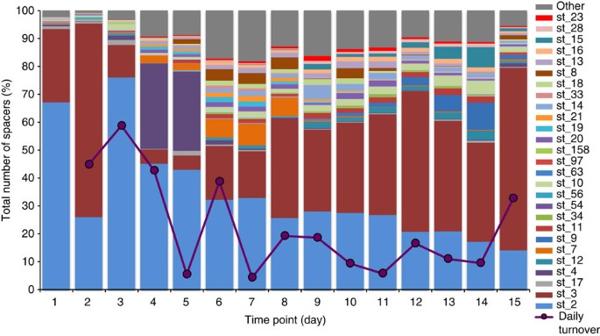Figure 3: Relative daily abundance of the most highly represented CRISPR1 spacers. The 27 spacers used in the analysis were identified as among the 10 most abundant spacers each day in the MOI2 experiment. The purple line indicates daily turnover in % spacer content. Figure 3: Relative daily abundance of the most highly represented CRISPR1 spacers. The 27 spacers used in the analysis were identified as among the 10 most abundant spacers each day in the MOI2 experiment. The purple line indicates daily turnover in % spacer content. Full size image Rates of shifts in bacterial sub-population abundances We defined sub-populations based on the spacer type acquired at the +1 location (the first newly acquired spacer, located on the leader end, following the wild-type repeat-spacer array). By tracking abundance patterns of specific +1 CRISPR1 spacers, we detected rapid oscillations in relative abundances of the sub-populations (for example, st_2 or st_3 at the +1 position in the MOI2 experiment; Supplementary Fig. S4 ). Interestingly, in the +2 or subsequent positions, only 16 of the 55 spacers were shared between the two sub-populations ( Supplementary Fig. S5 ). This indicates elevated, rapid and extensive diversification of the CRISPR complement is possible following acquisition of the first spacer, as host–phage populations co-evolve. Locus-based analysis of independent events To investigate bias in the proto-spacer representation, we counted the number of times that each specific spacer sequence derived from phage D2972 was sampled in a distinct event (Methods). Although one spacer type was sampled in 41 distinct events (st_4 in Fig. 4 ), 75% of all sampled spacers were represented by less than 10 events. Interestingly, 80% of st_4 acquisition events occurred during days 4 and 5. In contrast, for other spacers (for example, st_14, st_10, st_3), events accumulate progressively. 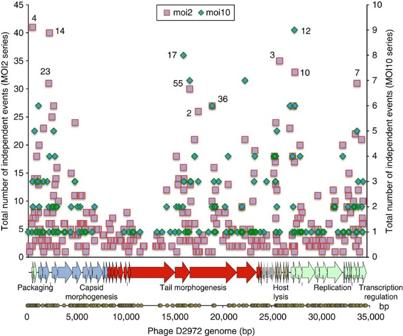Figure 4: Frequency of CRISPR1 spacer incorporation events sampled across phage D2972 genome. Most frequently sampled spacers (events) named with its spacer type number code plotted against the proto-spacer position in the phage D2972 genome (note there are two differentyaxes scales depend on the experiment). Thexaxis corresponds with D2972 phage genome location, predicted gene functions and transcription module (green, blue, red and brown for early, medium, late and late II transcribed genes, according to Duplessiset al.29). Location of the 233 perfect PAM (AGAAW) for CRISPR1 locus across the phage D2972 genome are indicated as olive dots underxaxis. Figure 4: Frequency of CRISPR1 spacer incorporation events sampled across phage D2972 genome. Most frequently sampled spacers (events) named with its spacer type number code plotted against the proto-spacer position in the phage D2972 genome (note there are two different y axes scales depend on the experiment). The x axis corresponds with D2972 phage genome location, predicted gene functions and transcription module (green, blue, red and brown for early, medium, late and late II transcribed genes, according to Duplessis et al. [29] ). Location of the 233 perfect PAM (AGAAW) for CRISPR1 locus across the phage D2972 genome are indicated as olive dots under x axis. Full size image Further, 9% of the 233 predicted proto-spacers were never represented, despite our analysis of 443,871 newly acquired CRISPR1 spacer sequences. We noted that most highly sampled spacers targeted five broad regions of the phage genome ( Fig. 5 ). This bias was also evident in terms of the total number of times a spacer was identified across the time series (overall spacer frequency). The same bias in phage genome targeting was evident in both experiments, and for both CRISPR–Cas systems, despite different PAMs for CRISPR1 and CRISPR3. 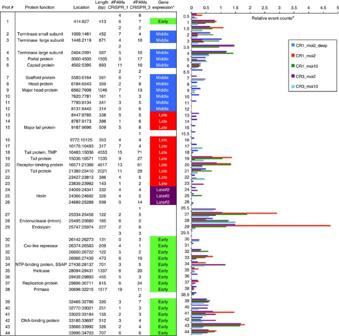Figure 5: Open reading frames (ORFs) in the genome of phage D2972 targeted by CRISPR1 and CRISPR3 spacers. Detailed information of ORFs in the genome of phage D2972. The predicted function, location of ORF, numbers of CRISPR1 and CRISPR3 PAMs numbers and expression module is shown along with the corresponding normalization to account for differences in sequencing depth (number of total spacers per sample), number of spacer events obtained per predicted protein (integer numbers) or inter-genic region (decimal numbers) and per number of perfect PAMs found in all the experiments (including a replicate for CRISPR1 MOI2, in blue) shown as#relative event counts. *Gene expression module according to Duplessiset al.29. Figure 5: Open reading frames (ORFs) in the genome of phage D2972 targeted by CRISPR1 and CRISPR3 spacers. Detailed information of ORFs in the genome of phage D2972. The predicted function, location of ORF, numbers of CRISPR1 and CRISPR3 PAMs numbers and expression module is shown along with the corresponding normalization to account for differences in sequencing depth (number of total spacers per sample), number of spacer events obtained per predicted protein (integer numbers) or inter-genic region (decimal numbers) and per number of perfect PAMs found in all the experiments (including a replicate for CRISPR1 MOI2, in blue) shown as # relative event counts. *Gene expression module according to Duplessis et al. [29] . Full size image Finally, tracking of lineages based on specific spacer incorporation events revealed the proliferation of early-rising sub-populations and the persistence of some strains over the time. Notably, we observed indications of sweeps, bottlenecks and fluctuations of the most-represented spacer types over time ( Fig. 6 ). 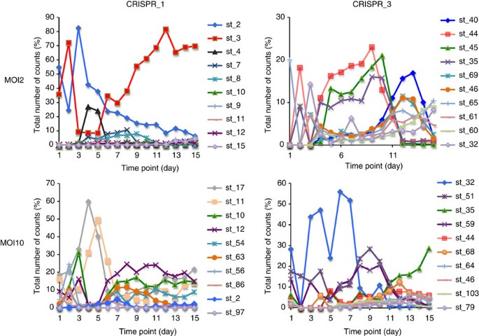Figure 6: Daily fluctuation of the 10 most-represented spacers for both CRISPR loci. Data from MOI2 and MOI10 experiments and normalized by the total number of counts per time point. Figure 6: Daily fluctuation of the 10 most-represented spacers for both CRISPR loci. Data from MOI2 and MOI10 experiments and normalized by the total number of counts per time point. Full size image Metagenomics has been used previously to characterize natural microbial communities, but has been rarely used to monitor experiments. The S. thermophilus DGCC7710 – phage D2972 co-culture serves as a model system for analysis of CRISPR locus dynamics. In our experiments (without previous selection), we detect a vast population diversity defined by the CRISPR spacer repertoire (a total of 3,256 distinct genotypes sampled). This is the first study documenting such diversity generated within an initially clonal population over a short time period. The identification of a migrant laboratory phage in the experiment suggests that PCR-based metagenomic analysis of CRISPR spacers could find application in discriminating among potential sources of a bacterial culture (for example, for tracking of biological agents). Daily turnover measurements indicate rapid evolution in the phage, presumably through escape mutation, a process necessary for phage survival in the face of rapid CRISPR spacer acquisition ( Figs 3 , 6 and Supplementary Figs S2, S3 and S4 ). One possible explanation for this over-representation of some spacer sequences is that some regions of the phage genome are more readily sampled by the CRISPR–Cas machinery than others. However, we ruled out phage ssDNA secondary structure, GC content and transcriptional patterns as potential explanations for the observed bias. We observed that some highly sampled phage regions were also targeted by wild-type spacers ( Supplementary Fig. S6 ), suggesting there is a link between existing immunity and novel spacer acquisition. Perhaps wild-type crRNA homologous to invasive DNA recruits the Cas machinery and drives novel spacer sampling from the target DNA [24] , consistent with priming of the CRISPR system by prior infection records [25] . Alternatively, some spacer sequences may be highly represented within the host population because they are strongly selected for. Similarly, under-represented spacers may be ineffective. Intriguingly, in both independent experiments, cells with a single +1 CRISPR1 spacer were more abundant than cells with additional spacers ( Supplementary Fig. S7 ). The higher abundance of cells with just one highly sampled spacer compared with cells with more spacers may also point to inequality in spacer value or a fitness cost associated with immunity build up. Transcription of multiple spacers would spread Cas protein complexes across CRISPR RNAs with varying affinities, reducing immunity compared with a single highly effective spacer. The possibility of ‘super’ spacer types or ‘super’ sensitive phage regions requires further investigation. Engineered strains using specific genotypes, with different combinations of highly efficient spacers or non-sampled spacers will shed light on this mechanistic issue. Model system S. thermophilus strain DGCC7710 was grown in a sterile 10% instant non-fat dry milk solution in diH 2 O, followed by incubation at 42 °C. After reaching stationary phase (7–8 h), 1% of the culture was used to re-inoculate fresh medium on a daily basis. In the co-culture host–phage challenges, bacteriophage D2972 was used, at multiplicities of infection of 10 and 2, with initial phage–host ratios of 10:1 and 2:1, respectively ( Supplementary Fig. S1 ). DNA sequencing of S. thermophilus CRISPR1 and CRISPR3 loci S. thermophilus genomic DNA of each time point was extracted according to Cremonesi et al. [26] , only altering the lysis solution (to raise pH) by adding NaOH before filtering. Before sequencing, both CRISPR1 and CRISPR3 loci were amplified by PCR with Pfu Ultra II Fusion HS DNA polymerase (Agilent Technologies) with the corresponding primers for each time point ( Supplementary Table S5 ), and purified twice using Ultra Clean PCR-purification columns (MoBio lab) and Qiaquick Gel Extraction (QIAGEN) from an agarose gel. Each PCR product was sequenced using 454 FLX Titanium high-throughput technology at W.M. Keck Center for Comparative and Functional Genomics (University of Illinois at Urbana-Champaign). Details of the number of sequences as well as spacers obtained per experiment, time point and locus, are described in Supplementary Table S1 . Determination of cell- and plaque-forming units Two samples of milk culture were taken to estimate total cell counts and phage counts for each time point. One culture sample was serially diluted in buffered peptone water and aliquoted onto pre-poured plates of “Man, Rogosa and Sharpe” agar (MRS) [27] for cell counts. The other culture sample was centrifuged (13,000 r.p.m., 7 min) and the resulting whey was used to make dilutions in buffered peptone water with 10 mM CaCl 2 . Spot titre plates were made by first growing DGCC7710 wild-type inoculating culture in MRS broth with 0.3% non-fat dairy milk to an optical density (OD 600 nm) of 0.2-0.5. The inoculating culture was then added at 10% to MRS soft agar with 10 mM CaCl 2 and dispensed on MRS pre-poured plates. Dilutions from the 10 mM CaCl 2 peptone water were spotted on the overlay. All plates were incubated overnight at 42 °C anaerobically. Detection of phage D2766 Regions of homology among the five phage genomes that flanked a heavily sampled region that were polymorphic were investigated. The primers derived from that strategy are located in position 25,037 (leader region) and 26,894 (reverse strand) in the corresponding D2972 genome. ACEphi1_fwd (5′-TCAACTCAAGGAGCAG-3′) and ACEphi1_rev (5′-CCATTACCTGTGCTTTTT-3′) were the pair of primers used to amplify the 1,857 bp polymorphic region. The primers were used on whey for several transfers within a PCR reaction containing also a high Pfu (Mastermix Polymerase) under the following PCR conditions: 95 °C/5 min, (95 °C/30 s, 47 °C/30 s, 72 °C/10 min) × 30 cycles, 72 °C/5 min. The resulting 3-kb amplicon was Sanger sequenced. Two sequences (amplicon too large to sequence across) were matched against our internal database of Streptococcus phage sequences, and showed 98.78% (forward) and 98.96% (reverse) identities to D2766. Computational analyses We developed a suite of tools for identifying and analysing CRISPR spacers from DNA-sequencing reads (described in detail in Sun et al. [28] ). We restate the procedure here briefly. The suite begins by identifying individual sequencing reads containing a repeat sequence of interest using a simple regular expression matching of the repeat sequence to all reads. It then inventories information about the order of the repeats and spacers on each read and then creates a database of the results. We grouped spacers based on those sharing 80% in length and 80% sequence identity to avoid over-representation of spacers derived of possible 454-sequencing errors. We call a grouping of 80% identity/80% length spacers a “spacer type”, and use these spacer types in the subsequent analysis. After processing all the reads for an experiment, a report is generated containing a summary of the unique spacer types and every configuration they are found in across the entire data set. For example, if a sequence contains the spacer types configuration A-B-C, it is treated as distinct from A-C-B, or A-B or A-C, and so on. Identification of spacers on reads is the basis for the following alignment step. See Sun et al. [28] for more details. For this study, we developed “Crispralign” to align CRISPR spacer types. As above, these types are based on the overlap of reads carrying spacers in the same order. Crispralign determines the frequency of each CRISPR spacer type and uses this frequency to assist in creating a simple alignment. For example, if the software encounters spacer type X with nothing preceding it, it searches the entire data set to see what spacer normally precedes X. If spacer type X was seen to follow spacer type Q twice and spacer type Z 10 times, then the script will assume spacer type Z was missing from this sequencing read and align spacer type F with those that following spacer type Z. Alternatively, if there is no clear prevalence seen in the entire data set for a particular spacer arrangement, gaps are introduced in the alignments and compared with other spacer types found in the sample. The Crispralign script and installation instructions can be downloaded here: https://github.com/kueda/crispalign . Accession codes : Sequencing data have been deposited in the NCBI Sequence Read Archive under the accession code SRA062737 . How to cite this article: Paez-Espino, D. et al. Strong bias in the bacterial CRISPR elements that confer immunity to phage. Nat. Commun. 4:1430 doi: 10.1038/ncomms2440 (2013).